Highly accelerated inverse electron-demand cycloaddition of electron-deficient azides with aliphatic cyclooctynes Strain-promoted azide–alkyne cycloaddition (SPAAC) as a conjugation tool has found broad application in material sciences, chemical biology and even in vivo use. However, despite tremendous effort, SPAAC remains fairly slow (0.2–0.5 M −1 s −1 ) and efforts to increase reaction rates by tailoring of cyclooctyne structure have suffered from a poor trade-off between cyclooctyne reactivity and stability. We here wish to report tremendous acceleration of strain-promoted cycloaddition of an aliphatic cyclooctyne (bicyclo[6.1.0]non-4-yne, BCN) with electron-deficient aryl azides, with reaction rate constants reaching 2.0–2.9 M −1 s −1 . A remarkable difference in rate constants of aliphatic cyclooctynes versus benzoannulated cyclooctynes is noted, enabling a next level of orthogonality by a judicious choice of azide–cyclooctyne combinations, which is inter alia applied in one-pot three-component protein labelling. The pivotal role of azide electronegativity is explained by density-functional theory calculations and electronic-structure analyses, which indicates an inverse electron-demand mechanism is operative with an aliphatic cyclooctyne. Recent years have seen a tremendous interest in a class of chemistry known as strain-promoted cycloadditions [1] . The high mutual reactivity of reaction components, yet (relative) inertness for a large repertoire of other molecular functionalities, explains the fast-growing popularity of strain-promoted cycloadditions for application in material sciences [2] , surface functionalization [3] , bioconjugation [4] , chemical biology and even in vivo use (known as bioorthogonal chemistry) [5] , [6] . The major focus in the field of strain-promoted cycloadditions—generally defined [1] as a bimolecular reaction of a strained system (typically an unsaturated carbocycle) with a complementary component (typically a 1,3-dipole or a diene)—has centred around cyclooctyne, the smallest stable cycloalkyne. Its reactivity with 1,3-dipoles, 1,3-dienes, carbenes and other functional groups has been reported throughout the years [1] , and inspired Bertozzi et al. [7] to develop strain-promoted alkyne–azide cycloaddition (SPAAC) as a copper-free version of the popular ‘click reaction’ for application in cellular assays and bioconjugation. Subsequently, a whole family of cyclooctynes has been developed ( Fig. 1 ), mostly with the aim to enhance the relatively slow reaction rate constant of plain cyclooctyne, for example, by introduction of electron-poor fluoride substituents as in difluorocyclooctyne (DIFO, 1 ) (ref. 8 ), or by dibenzoannulation as in dibenzocyclooctyne (DIBO, 2 ) (ref. 9 ). Dibenzo-aza-cyclooctyne (DIBAC, 3 ) first developed by us [10] , also called aza-dibenzocyclooctyne (ADIBO) [11] or dibenzocyclooctyne (DBCO) [12] displayed significantly enhanced reactivity and is currently the most broadly applied cyclooctyne for strain-promoted cycloadditions. Yet more reactive probes such as biarylazacyclooctynones (BARAC) [13] ( 4 ) and tetramethylthiacycloheptyne (TMTH) [14] ( 5 ) exist, but suffer from poor stability. Bicyclo[6.1.0]non-4yne (BCN, 6) is a stable, non-benzoannulated cyclooctyne that is synthetically readily accessible [15] , but generally regarded to be less reactive than DIBAC. Finally, Sondheimer diyne ( 7 ) is unique in the sense that it is able to react sequentially with two azides with distinctly different reaction rates [16] . In general it may be concluded that, despite tremendous synthetic effort, optimization of cycloaddition of azides with (stable) cyclooctynes has, depending on specific conditions, leveled off around 0.2–0.5 M −1 s −1 (refs 1 , 4 ). 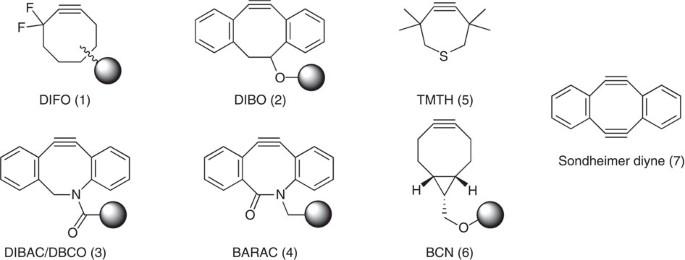Figure 1: Known cycloalkynes for bioconjugation. Cyclooctynes employed in strain-promoted alkyne–azide cycloaddition (SPAAC) most typically include DIBO (2), DIBAC (3) and BCN (6). Figure 1: Known cycloalkynes for bioconjugation. Cyclooctynes employed in strain-promoted alkyne–azide cycloaddition (SPAAC) most typically include DIBO ( 2 ), DIBAC ( 3 ) and BCN ( 6 ). Full size image We here wish to report tremendous acceleration of strain-promoted cycloaddition with cyclooctynes, only by modulation of the azide structure. In particular, it is found that BCN reacts with electron-poor aryl azides up to 29 times faster than with aliphatic azides, with reaction rate ratios reaching 2.0–2.9 M −1 s −1 . Moreover, a judicious choice of azide enables near-complete tailoring of BCN:DIBAC reaction rate ratios from 0.24 to >25, which is applied in the first orthogonal SPAAC reported to date. The remarkable difference in rate constants of aliphatic versus benzoannulated cyclooctynes, as well as the pivotal role of substituent electronegativity are explored and explained by density-functional theory (DFT) calculations [17] and electronic-structure analyses [18] . Azide–cyclooctyne structure–reactivity relationship Our investigations on the structure–reactivity relationship of azides in strain-promoted cycloadditions were stimulated by the fact that much effort has been devoted to the development of more reactive cyclooctynes [8] , [10] , [11] , [12] , [13] , [14] , [15] , but only scant information is available on the influence of the azide structure on SPAAC rates [19] , [20] . In addition, it struck us that SPAAC reaction rate constants are nearly always determined with an aliphatic azide (typically benzyl azide), but rarely with an aromatic azide. The reason to generally avoid aromatic azides for SPAAC presumably lies in the reported sevenfold reduced reactivity of phenyl azide in comparison with an aliphatic azide, at least in conjunction with DIBAC [19] . The observation that reaction rates of aromatic azides are hardly influenced by changing the electronic nature of substituents (as determined for p- methoxy and p- CF 3 -phenyl azide) [20] , has provided further ground to avoid aromatic azides for SPAAC. However, because an in-depth structure–reactivity relationship of azides with cyclooctynes is lacking to date, we designed a comparative study of aliphatic and aromatic azides in their reactivity with an aliphatic cyclooctyne (BCN) and a dibenzoannulated cyclooctyne (DIBAC). IR-based reaction rate determination To facilitate the evaluation of a large number of azides in reaction with cyclooctynes, the availability of a fast and straightforward method to follow conversion rates was desirable. However, the common nuclear magnetic resonance-based method for reaction rate determination is laborious and unsuitable for fast reactions ( k >1 M −1 s −1 ) as a consequence of the time-consuming data acquisition. An alternative method based on ultraviolet [21] , [22] is fast, but is also limited to cases where a difference exists in absorption between substrate(s) and product(s) at a specific wavelength. We reasoned that infrared (IR) detection should enable direct monitoring of substrate-to-product conversion, simply by integration of the distinct azide stretch vibration (around ±2,100 cm −1 ). Indeed, it was found that IR-monitoring of reactions performed in a 9:1 mixture of THF/H 2 O enables fast and accurate monitoring of azide disappearance, as exemplified for reaction of benzyl azide and BCN alcohol 6a ( Fig. 2a,b ; Supplementary Fig. 1 ). From this plot, a reaction rate constant of 0.07 M −1 s −1 could be readily derived ( Fig. 2c ; Supplementary Methods ). Other solvents were also explored, for example, 20% aqueous THF or pure MeOH, but in these cases signal-to-noise ratios were too small to measure azide stretch vibration. 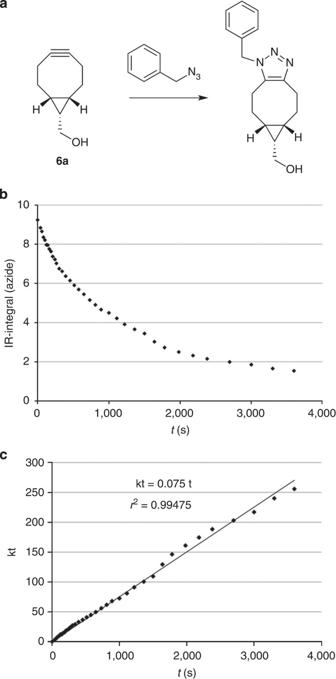Figure 2: Reaction rate determination based on IR. (a) Model SPAAC reaction between benzyl azide and non-functionalized BCN alcohol6a. (b) Data points collected by integration of N3stretch vibration of benzyl azide during reaction with BCN alcohol6a. (c) Determination of the second-order rate constantkfor the reaction of benzyl azide and BCN alcohol6aby linear regression. Figure 2: Reaction rate determination based on IR. ( a ) Model SPAAC reaction between benzyl azide and non-functionalized BCN alcohol 6a . ( b ) Data points collected by integration of N 3 stretch vibration of benzyl azide during reaction with BCN alcohol 6a . ( c ) Determination of the second-order rate constant k for the reaction of benzyl azide and BCN alcohol 6a by linear regression. Full size image Cycloadditions of azides with BCN or DIBAC Having established a practical protocol for the determination of reaction rate constants, a small range of aliphatic azides ( A – C , for synthesis see Supplementary Methods 2 ) was evaluated first ( Fig. 3 ; Table 1 , entries 1–3, and Supplementary Table 1 ). Not surprisingly, near-identical rate constants were determined for azides A – C in reaction with BCN alcohol ( 6a ) or with a DIBAC derivative ( 3a ). Similar to earlier reported data [10] , [15] , an approximately three- to fourfold higher reactivity was observed for DIBAC versus BCN (k BCN :k DIBAC ). It must be noted, however, that the absolute rate constants as measured by this protocol are about twofold lower than those reported earlier in other solvent systems [1] . One sensible explanation lies in the fact that 1,3-dipolar cycloadditions generally proceed faster in a more polar environment (for example, 50% aqueous CH 3 CN) [23] , as for example was also demonstrated by us for strain-promoted nitrone cycloadditions [24] . Indeed, competition experiments in a 2:1 mixture of CD 3 CN/D 2 O ( Supplementary Methods 5 ) indicate k values (numbers in brackets) that are a factor 1.5–2.5 higher than those obtained by IR in 9:1 THF/H 2 O. 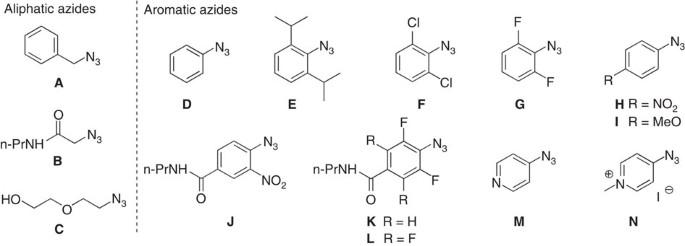Figure 3: Azide structure determines reaction rate. Structures of aliphatic (A–C) and (substituted) aromatic (D–N) azides. Figure 3: Azide structure determines reaction rate. Structures of aliphatic ( A – C ) and (substituted) aromatic ( D – N ) azides. Full size image Table 1 Experimentally determined absolute (M −1 s −1 ) and relative rate constants (BCN 6a versus DIBAC 3a ) for SPAAC with azides A - N . Full size table The first unexpected result was obtained while determining the rate constants for phenyl azide ( D , entry 4). While the sevenfold drop in reactivity with DIBAC was in line with earlier observations [19] , [20] , reaction with BCN unexpectedly proceeded 2.9 × faster in comparison with benzyl azide ( A , entry 1). Thus, in a side-by-side comparison, reaction of phenyl azide with BCN is in fact 6 × faster than with DIBAC, quite opposite to aliphatic azides. Stimulated by this finding, we were curious to investigate whether cycloaddition of BCN with 2,6-diisopropylphenyl azide ( E ) would be further accelerated, as reported for Sondheimer diyne 7 (ref. 20 ). However, in this case, only a modest effect was observed (1.5 × faster than unsubstituted phenyl azide, D ), while DIBAC, a dibenzoannulated cyclooctyne, like Sondheimer diyne, showed a large increase in reaction rate (23 × faster). Puzzled by these contradictory results, a range of substituted aryl azides ( F – N ) was subsequently synthesized ( Supplementary Methods 2 ) and evaluated in reaction with BCN and DIBAC (entries 6–14). It was found that replacing the o- isopropyl groups with a less sterically hindered but more electronegative halogen group (Cl or F) was favourable for the reaction with BCN, but not for DIBAC. The positive effect of an electronegative substituent on reactivity with BCN was also established for p- nitrophenyl azide ( H , entry 8), but quite opposite for reaction with DIBAC, thereby reaching a BCN:DIBAC reactivity ratio of a factor 27. Entries 9 and 10 further underline the positive correlation between electronegativity and cyclooaddition reactivity for BCN, but not for DIBAC. Finally, four particularly electron-poor aryl azides ( K – N ) were evaluated in a reaction with BCN and DIBAC (entries 11–14). Much to our delight, N -propyl 4-azido-2,3,5,6-tetrafluorobenzamide ( L , entry 12) and 4-azido-1-methylpyridinium iodide ( N , entry 14) reached reaction rate constants of 1.23 and 2.0 M −1 s −1 (or 2.9 M −1 s −1 by extrapolation from the competition experiment, Supplementary Methods 5 ), respectively, the highest absolute number for SPAAC (with a stable cycloalkyne), as well as relative BCN-to-DIBAC ratio (40 × faster) reported to date. Frontier molecular orbital considerations The marked increase in reaction rate for electron-poor azides is in sharp contrast to earlier findings of studies focusing on the influence of electron-withdrawing substituents on SPAAC, all of which have been suggestive of a HOMO azide –LUMO cyclooctyne interaction. For example, Hosoya et al. noted a 3.9 × increase in reaction rate for p- MeOC 6 H 4 N 3 ( I ) versus PhN 3 in reaction with 7 (ref. 20 ). A positive effect on reactivity (1.6 × faster) upon cyclooctyne fluorination, as in DIFO [8] or BARAC [25] , or upon DIBAC halogenation (up to 2.2 × faster) [26] further supports this notion. Interestingly, the fast reaction of electron-poor azides with an aliphatic cyclooctyne (BCN) as reported here is highly indicative of an alternative frontier orbital interaction. Further experimental support for the latter hypothesis is found in the much faster reaction of cyclooctyne 8 ( Supplementary Methods 3 ) with p- nitrophenyl azide than with benzyl azide (6 × faster), while only a negligible reaction rate difference was noted for the more electron-deficient cyclooctyne 9 ( Fig. 4 ). 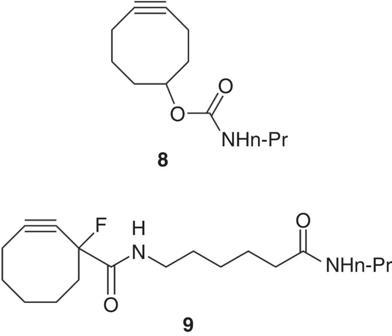Figure 4: Cyclooctyne structures determines reaction rate. Structures of a regular cyclooctyne8and an electron-poor cyclooctyne9as used in a competition experiment betweenp-NO2C6H4N3(H) and benzyl azide (A). Figure 4: Cyclooctyne structures determines reaction rate. Structures of a regular cyclooctyne 8 and an electron-poor cyclooctyne 9 as used in a competition experiment between p -NO 2 C 6 H 4 N 3 ( H ) and benzyl azide ( A ). Full size image Our relativistic DFT calculations [17] (at ZORA-OLYP/TZ2P, Supplementary Methods 8 ) [27] , [28] , [29] confirm the above reactivity trend of the reactions involving BCN (see Supplementary Table 2–4 for full structural and energy details). Thus, the barrier E a for the reaction of BCN with A , D , E , F and G decreases monotonically from 16.9 to 14.4 kcal mol −1 as the rate constant increases from 0.07 to 0.63 M −1 s −1 (see Table 2 ). The formation of the new C–N bonds occurs in an asynchronous manner: in the transition state, the bond length d 2 involving the aryl- or alkyl-substituted azide nitrogen runs somewhat behind that ( d 1 ) involving the other nitrogen atom. All reactions are pronouncedly exothermic with reaction energies E r between −55 and −60 kcal mol −1 . Table 2 Quantum-chemically computed key parameters of selected SPAAC reactions for BCN*. Full size table Interestingly, the DFT computations reveal that these fast cycloadditions with electron-poor azides proceed via an inverse electron-demand SPAAC mechanism (IED SPAAC). This is in line with the fact that BCN undergoes extremely fast IED Diels–Alder cycloaddition with 1,2,4,5-tetrazines [20] , [30] , [33] , while DIBAC is inert [31] . Fig. 5 is a schematic representation of the frontier molecular orbital interactions between the BCN and phenyl azide reactants in the transition state that emerge from our quantitative Kohn–Sham electronic-structure analyses. Activation-strain analyses [32] confirm that the overall orbital interactions indeed contribute ca −35 kcal mol −1 of stabilization, but that net interactions between the reactants in the TS are small, at most −0.8 kcal mol −1 , due to substantial Pauli repulsion between closed-shell orbitals on each of the two fragments. The dominant donor–acceptor orbital interactions are between the π electrons of BCN and the relatively low-energy LUMO of the azide. The associated ‘inverse’ HOMO BCN –LUMO azide gap of 1.8–2.4 eV is in all cases significantly smaller than the ‘normal’ HOMO azide –LUMO BCN gap of 4.5–4.9 eV (see Table 2 ). Besides the in-plane HOMO of BCN and azides, also the corresponding perpendicular π orbitals located on the BCN triple bond and azide N 3 moiety, respectively, contribute to the donor–acceptor interactions (see Fig. 5 ). The inverse electron donation from BCN HOMO and HOMO–1 to the azide is significantly larger, 0.22–0.26 electrons, than the normal electron donation from azide HOMO and HOMO–2 (or HOMO–3) to BCN, 0.07–0.10 electrons (not shown in Table 2 ). This agrees with the smaller inverse HOMO–LUMO gap and confirms the predominant IED character of azide with aliphatic cyclooctynes. 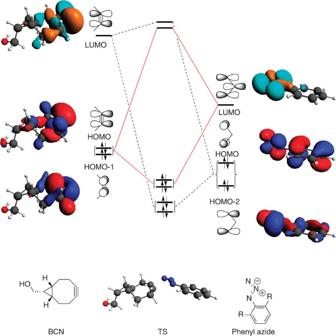Figure 5: Frontier orbital interactions in SPAAC or IED SPAAC. Schematic representation of the BCN–azide frontier molecular orbital interactions emerging from our quantitative Kohn–Sham electronic-structure analyses. Figure 5: Frontier orbital interactions in SPAAC or IED SPAAC. Schematic representation of the BCN–azide frontier molecular orbital interactions emerging from our quantitative Kohn–Sham electronic-structure analyses. Full size image One-pot three-component cycloadditions by orthogonal SPAAC Finally, the high reactivity of DIBAC and BCN with aliphatic or (electron-poor) aromatic azides, respectively, opens up the unique possibility of orthogonal SPAAC with two azides. First, we subjected 2,6-difluorophenyl azide derivative K to an excess of BCN alcohol 6a and a DIBAC derivative 3b (five equiv. each, Supplementary Fig. 2 ) in CD 3 CN/D 2 O (3:1). As expected, analysis of the crude reaction mixture with 1 H nuclear magnetic resonance led to the sole detection of the (3+2) cycloadduct formed by reaction with BCN, but no DIBAC-derived triazole ( Supplementary Fig. 10 ). A further level of selectivity was attained by mixing compound 10 ( Fig. 6 ), bearing one aliphatic and one electron-deficient aryl azide, with a twofold excess of BCN alcohol 6a and DIBAC derivative 3c ( Supplementary Fig. 3 ; Supplementary Methods 6 ), which led to the formation of a mixed BCN,DIBAC-bistriazole ( 12 ) as a pure compound in 83% yield after silica gel column chromatography, with only minor amounts ( ≪ 6%) of double-addition products of 10 with BCN or DIBAC ( Supplementary Fig. 23 ). The concept of a judicious choice of azide–cyclooctyne combination for orthogonal SPAAC was finally extended to a biological context by simultaneous incubation of green fluorescent protein (GFP) bearing a genetically encoded BCN [33] ( Fig. 6 ) with stoichiometric 10 and DIBAC-TAMRA ( 3d , Supplementary Methods 7 ). The reaction mixture was analysed by protein gel electrophoresis and in-gel fluorescence detection ( Supplementary Fig. 4 ). Incubation with 10 led to efficient labelling in only 2 h, while only minor labelling was observed upon similar incubation with bis-azido-triethylene glycol reagent 11 . In this respect, the here presented one-pot sequential SPAAC for labelling of a BCN-bearing protein bears resemblance, yet is nicely complementary, to the procedure reported by Hosoya et al. [16] for three-component labelling of an azido-bearing protein in the presence of Sondheimer diyne and an azido-fluorophore. 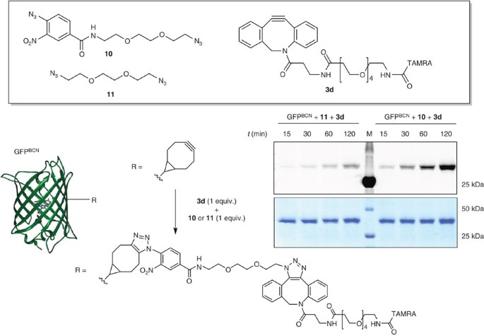Figure 6: Judicious choice of cyclooctyne-azide combination enables selective SPAAC. Labeling of GFPBCN(20 μM, 37 °C) with stoichiometric DIBAC-TAMRA (3d) in the presence of a bivalent linker containing either aliphatic and aromatic azide10or two aliphatic azides11shows significantly more labeling with linker10than with11. Figure 6: Judicious choice of cyclooctyne-azide combination enables selective SPAAC. Labeling of GFP BCN (20 μM, 37 °C) with stoichiometric DIBAC-TAMRA ( 3d ) in the presence of a bivalent linker containing either aliphatic and aromatic azide 10 or two aliphatic azides 11 shows significantly more labeling with linker 10 than with 11 . Full size image In conclusion, it was established that aliphatic and aromatic azides display a striking difference in reactivity, with strong preference for benzoannulated and aliphatic cyclooctynes, respectively. The latter experimental finding is strongly supported by relativistic DFT calculation, which indicate that aromatic azides and aliphatic cyclooctynes (in particular BCN) react via an IED mechanism, with the dominant donor–acceptor orbital interactions involving the π electrons of BCN (HOMO) and the LUMO of the azide, opposite to what currently is assumed to be the operative mechanism during SPAAC. The latter mode of reactivity enabled the development of highly accelerated SPAAC by means of introduction of electron-withdrawing substituents on the aromatic azide, thereby leading to unprecedented reaction rates (>2 M −1 s −1 ), up to 30-fold faster than ‘traditional’ SPAAC. In this respect, use of IED SPAAC also compares favourably with the so-called supersensitive copper-catalysed click chemistry, which can be accelerated only 4–6 times by including picolyl azides instead of regular benzyl azides [34] , [35] . It must be noted that several research groups reported on a sizable effect of electronegative substituents on aryl azides in cycloaddition with alkenes already 50 years ago [23] , [36] , [37] . For example, an approximate fourfold reaction rate enhancement was reported by Nowack et al. for nitro-substituted versus unsubstituted phenyl azide in reaction with norbornene [36] . Even more markedly, picryl azide was found to react with norbornene almost 1,000 times faster than phenyl azide, which is even further enhanced in reaction with electron-rich vinyl ethers and enamines as reported by Bailey and White [37] . The latter phenomenon was investigated in-depth by Huisgen et al. [23] and it was proposed that electronegative aryl substituents are able to lower the energy of the (concerted) transition state in cycloaddition with electron-rich olefin-like enamines by partial (negative) charge delocalization. However, why such a substituent effect is also operative in cycloaddition with neutral alkenes (for example, norbornene) and why the effect is so much smaller for alkenes with an electron-withdrawing substituent, remains unexplained. The current study first of all reports absolute reaction rate constants for cycloaddition with BCN that are significantly faster than those reported for alkenes, for example, a factor 1,000 times higher than for norbornene [23] . Moreover, a similar Hammett effect in reaction with alkynes was to the best of our knowledge unexplored to date. Furthermore, we have elucidated the bonding mechanism between the reactants in terms of quantitative Kohn–Sham molecular orbital theory based on DFT computations. These analyses link the reactivity trend of our SPAAC reactions involving BCN to the ‘inverse’ HOMO BCN –LUMO azide gap. We are confident that the latter insight will provide solid ground for the design of yet faster strain-promoted cycloadditions. A practical convenience of the IED reactions reported herein furthermore lies in the fact that BCN and several of the aromatic azides are readily synthesized or commercially available, such as, for example, photoaffinity labelling reagents based on azidotetrafluorobenzoic acid [38] . It is clear that the reaction rate constants of the here presented accelerated IED SPAAC still lag far behind those involved with IED cycloadditions of tetrazines. [1] , [4] , [22] , [30] However, besides specific in vivo applications that proceed at extremely small concentrations, in the vast majority of circumstances such high reaction rates as pertaining to tetrazine ligation are not a prerequisite. Hence, also given the high popularity of (copper-free) click chemistry, broad application of the here reported accelerated SPAAC may be foreseen, in scientific areas spanning from polymer and materials science, chemical and cell biology and beyond. Furthermore, it is to be expected that with growing understanding of IED SPAAC, even faster probes may be readily designed in forth-coming years. Efforts in this direction, as well as further computational analyses with the aim to more rationally design IED SPAAC, are currently under investigation in our laboratories. How to cite this article : Dommerholt, J. et al. Highly accelerated inverse electron-demand cycloaddition of electron-deficient azides with aliphatic cyclooctynes. Nat. Commun. 5:5378 doi: 10.1038/ncomms6378 (2014).